The evolution of sensory divergence in the context of limited gene flow in the bumblebee bat The sensory drive theory of speciation predicts that populations of the same species inhabiting different environments can differ in sensory traits, and that this sensory difference can ultimately drive speciation. However, even in the best-known examples of sensory ecology driven speciation, it is uncertain whether the variation in sensory traits is the cause or the consequence of a reduction in levels of gene flow. Here we show strong genetic differentiation, no gene flow and large echolocation differences between the allopatric Myanmar and Thai populations of the world's smallest mammal, Craseonycteris thonglongyai , and suggest that geographic isolation most likely preceded sensory divergence. Within the geographically continuous Thai population, we show that geographic distance has a primary role in limiting gene flow rather than echolocation divergence. In line with sensory-driven speciation models, we suggest that in C. thonglongyai , limited gene flow creates the suitable conditions that favour the evolution of sensory divergence via local adaptation. Theoretical models [1] , [2] and a few empirical studies [3] , [4] have suggested the role of divergent ecology and sensory perception in speciation. Despite classical studies investigating the role of sensory ecology in speciation, [3] , [5] it has not yet been possible to confirm whether sensory divergence is initially responsible for limiting gene flow or results as a consequence of limited gene flow [6] . Typically, most classical research on speciation follows a retrospective 'spyglass' approach, whereby the causes and mechanisms of speciation are inferred retrospectively after the speciation process is finished [7] . Although this approach has undeniably improved our understanding of speciation, it often lacks resolution at the early stages of the process, either because after speciation is completed, the signal has been confounded by post-speciation changes or simply because of the lack of historical ecological and/or behavioural data when the process was initiated [8] . Templeton [9] suggested that 'The closer to the speciation process, the greater the ability to focus upon the genetics of speciation', leading to the view that research is needed at the population/species interface to uncover how speciation occurs [7] , [8] , [10] . Therefore, studying the population/species interface, using a 'magnifying glass' approach, can reveal important aspects of speciation and how ecology, behaviour and genetics interact in different situations to cause the evolution of barriers to gene flow [7] , [11] , particularly important in the case of sensory ecology driven speciation. The majority of bats use sound (echolocation) to orient themselves in their environment, locate their food and communicate [12] . A bat's echolocation signal and its ability to perceive this signal are functionally linked, as the bat must be physically able to hear the echoes of its outgoing calls [13] . Therefore, studying the signal or echolocation call in bats will inform our understanding of their sensory system and perception capabilities [11] , [13] . Currently the genetic mechanisms that control echolocation are being uncovered and studies are starting to explore the role that echolocation has in communication and sexual selection [14] . Recent studies have suggested that changes in echolocation frequency (for example, Rhinolophus ) are associated with assortative mating, reproductive isolation and ultimately speciation, regardless of external barriers to gene flow [5] . Therefore, bat species are an excellent mammalian model to study the role of sensory drive (that is, echolocation calls) in the speciation process [11] , [15] . One such species is Craseonycteris thonglongyai , a rare and endangered, charismatic bat species, considered as the World's smallest mammal and restricted to a 2,000-km 2 region that straddles the Thai–Myanmar border [16] . Currently, the Thai and Myanmar populations are disjointed, although the long-term presence of suitable intervening karst landscape suggests that this may once have been a continuous distribution ( Fig. 1 ). Despite being morphologically indistinguishable [17] , observed variation in echolocation calls between Thailand [18] and Myanmar [19] suggested that more than one species might be present. Therefore, studying both the allopatric and sympatric populations offers a unique opportunity to study the factors that influence population structure, gene flow and sensory trait's divergence across an entire species range and at different evolutionary timeframes. 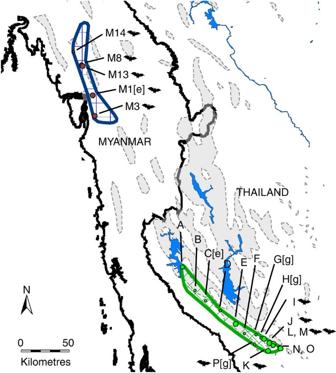Figure 1: Map of 21 colonies whereC. thonglongyaiwere sampled and recorded. Grey shaded areas represent limestone areas and blue shaded areas represent inland water bodies (dams).C. thonglongyaidistribution in Thailand (green) and Myanmar (dark blue) were taken from Puechmailleet al.16A bat is represented next to each site whereM. siligorensiswas recorded. Myanmar colonies are labelled as M1, M3, M8, M13 and M14. Thailand colonies are labelled A–P. [e] indicates a colony where only echolocation data were recorded, while [g] designates a colony with only genetic data. Figure 1: Map of 21 colonies where C. thonglongyai were sampled and recorded. Grey shaded areas represent limestone areas and blue shaded areas represent inland water bodies (dams). C. thonglongyai distribution in Thailand (green) and Myanmar (dark blue) were taken from Puechmaille et al . [16] A bat is represented next to each site where M. siligorensis was recorded. Myanmar colonies are labelled as M1, M3, M8, M13 and M14. Thailand colonies are labelled A–P. [e] indicates a colony where only echolocation data were recorded, while [g] designates a colony with only genetic data. Full size image Here we used both a 'spyglass' and 'magnifying glass' approach to untangle the early drivers of speciation in allopatric and sympatric populations of C. thonglongyai , the sole representative of the monotypic bat family Craseonycteridae. To illuminate the early stages of the speciation process, we examined the ecological and genetic factors that could have limited gene flow and driven local adaptation in these unique populations. We specifically focus on the role that echolocation has in this process. We show that currently no gene flow is occurring between the geographically isolated allopatric populations in Thailand and Myanmar, and infer that geographic isolation most likely preceded the echolocation divergence. Within the sympatric populations in Thailand, we identified geographic distance rather than echolocation divergence as the major factor shaping population structure across the entire range. We suggest that echolocation divergence within Thailand, most likely resulting from interspecific competition, evolved in a context of limited gene flow, which itself resulted from the extreme localized dispersal of this species. The spyglass approach To reconstruct the spatio-temporal history of these populations and determine the role that echolocation call variation may have in speciation, we generated and analysed a multi-genic data set (Cytochrome b and partial D-loop, X- and Y-introns and microsatellites; GenBank accession no. GU247601–247751, Supplementary Tables S1 and S2 ) and collected acoustic data from throughout the species' range ( Fig. 1 ). Intensive trapping, sampling and acoustic recording were carried out in Thailand and Myanmar ( Fig. 1 ). These data confirmed the marked and significant difference in echolocation calls between Thailand and Myanmar (Thailand: N =4,188, 70.125–79.875 kHz and Myanmar: N =1,472, 76.875–83.625 kHz, generalized linear mixed model, P =0.002; Fig. 2a ; Supplementary Fig. S1 ). Bayesian phylogenetic analyses based on a 1.8-kb mitochondrial fragment of 602 samples and two different NUMTs (mitochondrial pseudogenes) showed that the Thai and Myanmar populations were reciprocally monophyletic with a posterior probability of 1.00 ( Fig. 2b ). This clear Thai–Myanmar split was confirmed at the nuclear level by screening all individuals ( n =659) for 15 microsatellites ( F st =0.49, P <0.001; Fig. 2c–d ) and five nuclear single-nucleotide polymorphisms (SNPs), which showed almost complete lineage sorting ( Supplementary Fig. S2 ). The overall strong differentiation of all markers investigated combined with the complete lineage sorting of the mitochondrial fragment ( Fig. 2b ), two nuclear SNPs ( Supplementary Fig. S2 ) and the absence of shared alleles at one microsatellite locus, strongly advocate for a total absence of gene flow between the allopatric Thai and Myanmar populations. Relying on the molecular clock, the split between the two populations is dated to approximately 0.4 Mya (95% highest probability density, 0.268–0.545 Mya). Genetic diversity indices of the Myanmar population are significantly reduced at the mitochondrial (Thailand, Hs=0.92; Myanmar, Hs=0.36; permutation test, P =0.006) and nuclear (Thailand, Hs=0.56; Myanmar, Hs=0.43; permutation test, P =0.014) levels compared with the Thai population. Similarly, nucleotide diversity of the mitochondrial DNA fragment calculated per site in Thailand and Myanmar differ strongly with more than 10-fold differences (Thailand: average π =0.0034, min–max: 0.0028–0.0048; Myanmar: average π =0.00027, min–max: 0.00013–0.00050), indicating that the Myanmar population probably originated from a small number of individuals, either as a consequence of a strong bottleneck or more likely via a founder effect. However, to fully elucidate whether echolocation variation drove the isolation of the two populations or evolved after their split requires knowledge about distribution of species and the echolocation frequency of the population at the time of divergence. As this is not available, we turned to the sympatric Thai population to address this question. 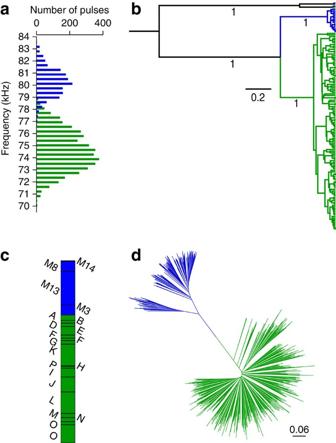Figure 2: Distinction between Thailand and Myanmar populations. (a) Distribution of echolocation calls recorded in Thailand (green;n=4,188) and Myanmar (blue;n=1,472). (b) Bayesian phylogenetic tree based on a 1.8-kb mitochondrial fragment of 602 samples and two different NUMTs (mitochondrial pseudogenes) showing the monophyly of the Thai (green) and Myanmar (blue)C. thonglongyai. The tree is rooted with two distinct NUMTs found in both populations. Bayesian posterior probabilities are shown below branches of interest. (c) Graphical representation of 196 Myanmar and 463 Thai individuals according to their probability to belong to each of the two clusters defined by STRUCTURE (black lines separate individuals sampled at different colonies). (d) Neighbour-Joining tree showing the relationships between 196 Myanmar (in blue) and 463 Thai (in green) individuals based on 15 microsatellites (Da distance). Figure 2: Distinction between Thailand and Myanmar populations. ( a ) Distribution of echolocation calls recorded in Thailand (green; n =4,188) and Myanmar (blue; n =1,472). ( b ) Bayesian phylogenetic tree based on a 1.8-kb mitochondrial fragment of 602 samples and two different NUMTs (mitochondrial pseudogenes) showing the monophyly of the Thai (green) and Myanmar (blue) C. thonglongyai . The tree is rooted with two distinct NUMTs found in both populations. Bayesian posterior probabilities are shown below branches of interest. ( c ) Graphical representation of 196 Myanmar and 463 Thai individuals according to their probability to belong to each of the two clusters defined by STRUCTURE (black lines separate individuals sampled at different colonies). ( d ) Neighbour-Joining tree showing the relationships between 196 Myanmar (in blue) and 463 Thai (in green) individuals based on 15 microsatellites (Da distance). Full size image The magnifying glass approach As the first steps of speciation occur at the population/species interface [7] , [8] , [9] , [20] , we investigated the recent spatio-temporal history of the Thai population and the relationship between genetic structure and echolocation frequency at the population level. To investigate past changes in distribution, we assessed whether the Thai population has been stable, increased in size (demographic expansion) or spatially expanded (spatial expansion) [21] using mismatch distribution analyses of mitochondrial fragments ( n =462). A model of stable population size was rejected for all Thai colonies (non-overlapping 99% confidence intervals of θ 0 and θ 1 , two mutation parameters that are related to the effective size of the population before and after a putative expansion, respectively). While the Southern Thai colonies (H, I, J and L, M, N, O, Fig. 1 ) fitted both models of demographic and spatial expansion equally well, the Central (E, F and G, Fig. 1 ) and Northern colonies (A, B and D, Fig. 1 ) fitted a model of spatial expansion but not a model of pure demographic expansion ( Supplementary Fig. S3 ). Principal component analysis of microsatellite data showed a strong population structure orientated along the Northwest–Southeast direction ( Fig. 3a–d ). This structure was confirmed by a Mantel test showing a very strong correlation between geographic and genetic distances (Mantel test; r =0.95, R 2 =0.90, P <0.001; Fig. 3e ). This strong correlation could theoretically result from different evolutionary histories such as secondary contact between two previously isolated populations or spatial expansion from a single population. Although the secondary contact scenario cannot be excluded, mismatch distributions do not support the presence of two isolated populations, but rather suggest that a single population was most likely present in the Southern part of their range and recently expanded northwards. Analyses that simulate the Thai population spatially expanding under a wide range of migration rate and population growth rate show that the strong isolation by distance pattern observed ( Fig. 3e ) can result from a recent spatial expansion when gene flow is restricted to neighbouring populations ( Supplementary Table S3 and Fig. S4 ). The average dispersal distance estimated from the slope of the regression between genetic distance and geographic distance was 2.2–5.7 km, indeed demonstrating extreme localized dispersal. 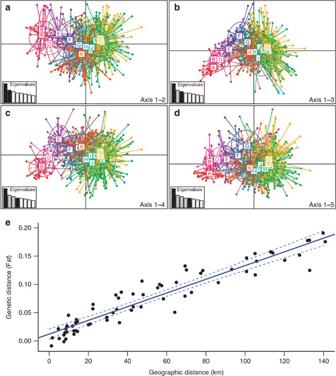Figure 3: Population structure within Thailand. Principal component analysis (PCA) showing the population structure of individuals orientated along the Northwest–Southeast direction with the first axis (explaining 8.46% of the variance) versus the (a) second axis (5.56%), (b) third axis (4.97%), (c) fourth axis (4.34%) and (d) fifth axis (4.24%). For each graph, the inset represents the eigenvalues of the two axes. Individuals from each of the 14 colonies are represented in different colours, and the colonies range from A in the Northwest to O in the Southeast. Colony P was excluded from the PCA, as only single individual was available from this site. (e) Relationship between genetic distance (Fst) versus geographic distance for the 12 colonies with echolocation and genetic data in Thailand (n=442 individuals). Significance was tested using a Mantel test (r=0.95,R2=0.90,P<0.001). Figure 3: Population structure within Thailand. Principal component analysis (PCA) showing the population structure of individuals orientated along the Northwest–Southeast direction with the first axis (explaining 8.46% of the variance) versus the ( a ) second axis (5.56%), ( b ) third axis (4.97%), ( c ) fourth axis (4.34%) and ( d ) fifth axis (4.24%). For each graph, the inset represents the eigenvalues of the two axes. Individuals from each of the 14 colonies are represented in different colours, and the colonies range from A in the Northwest to O in the Southeast. Colony P was excluded from the PCA, as only single individual was available from this site. ( e ) Relationship between genetic distance (F st ) versus geographic distance for the 12 colonies with echolocation and genetic data in Thailand ( n =442 individuals). Significance was tested using a Mantel test ( r =0.95, R 2 =0.90, P <0.001). Full size image The geographically continuous Thai population showed an abrupt change in echolocation frequency between colonies having similar echolocation calls (range: 73.35–73.96 kHz) for over 100 km in the Northern/Central part of their range and then a sudden increase ( ∼ 3 kHz) in <20 km in the Southern part ( Fig. 4 ). As body size and echolocation frequency are correlated across species [22] , we used forearm length as a proxy of body size and showed that body size differences are unlikely to explain the observed echolocation difference (Spearman's rank correlation, ñ =−0.17, P =0.53). We then used causal modelling on resemblance matrices [23] , [24] to investigate the combination of factors driving genetic differentiation between colonies. We first evaluated the set of diagnostic statistical tests of the seven possible organizational models, which included geographic distance, the presence of barriers (areas without limestone), echolocation distance (measured by the absolute echolocation difference) and genetic distance (measured by the F st index calculated on 14 microsatellites; Supplementary Information ). Only one organizational model, which included geographic distance, echolocation distance and genetic distance, was fully supported by all statistical expectations ( Supplementary Table S4 ). The six possible models of causal relationships between geographic distance, echolocation distance and genetic distance were then compared with the predictions of the models [23] . Five models were not supported by the data, as one or several of their predictions were not realized ( Supplementary Table S5 ), while one model was fully supported. This latter model supports the primary influence of geographic distance on genetic distance, which itself influences echolocation distance. 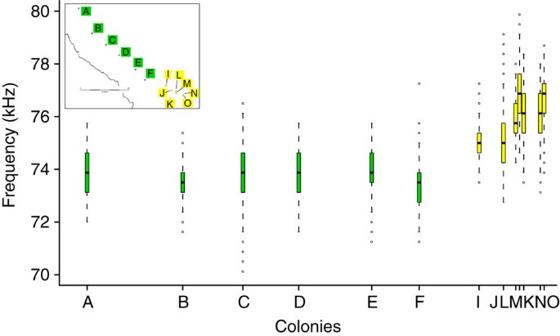Figure 4: Echolocation call variation within Thailand. Graph showing the variation in frequency of free flyingC. thonglongyairecorded at different colonies represented on the inset map. Colonies are arranged on theXaxis according to their score at the first axis (explaining 98.9% of the variance) of a principal component analysis on their geographic coordinates (latitude, longitude). For each boxplot, the box represents the 0.25 quantile, median and 0.75 quantile. On either side of the box, the whiskers extend to the minimum and maximum. To showcase possible outliers, whiskers were shortened to a length of one time the box length. The colours in the plot correspond to the colours in the inset map. Figure 4: Echolocation call variation within Thailand. Graph showing the variation in frequency of free flying C. thonglongyai recorded at different colonies represented on the inset map. Colonies are arranged on the X axis according to their score at the first axis (explaining 98.9% of the variance) of a principal component analysis on their geographic coordinates (latitude, longitude). For each boxplot, the box represents the 0.25 quantile, median and 0.75 quantile. On either side of the box, the whiskers extend to the minimum and maximum. To showcase possible outliers, whiskers were shortened to a length of one time the box length. The colours in the plot correspond to the colours in the inset map. Full size image Echolocation and drift To investigate if this change in echolocation could result from echolocation drift, we assessed the short- and long-term population sizes in the North/Centre and South of Kanchanaburi. We used the actual average colony size [16] as a proxy for short-term population size, and mitochondrial and nuclear genetic diversity found within colonies as a proxy for long-term population size; high genetic diversities are being associated with large effective population sizes and reduced drift, whereas low genetic diversities are being associated with reduced population sizes and increased drift [25] . The actual average colony size (South: 275; North/Centre: 248) did not significantly differ between Northern/Central and Southern colonies (Wilcoxon Mann–Whitney rank-sum test, n =20, P =0.19). A one-sided permutation test showed that the Northern/Central colonies had significantly reduced mitochondrial (North/Centre, Hs=0.87; South, Hs=0.94; P =0.01) and nuclear (North/Centre, Hs=0.52; South, Hs=0.57; P =0.04) gene diversities when compared with the Southern colonies. These short-term and long-term population sizes suggest that the Northern/Central colonies, which most likely spatially expanded, were equally or more prone to drift than the Southern colonies, and therefore, if drift had a role in echolocation frequency change, the Northern/Central colonies should show similar or higher variation across colonies than their Southern counterparts. Contrary to this expectation, C. thonglongyai in the Northern/Central part of the range shows little echolocation variation over 100 km (colonies A to F, Fig. 4 ). Therefore, this observation of a nonrandom pattern of echolocation call variation ( Fig. 4 ) supports the view that variation in echolocation within the Thai population may have resulted from adaptation as opposed to drift. Echolocation and genomic selection There are marked differences in echolocation call between the North/Centre and South of Kanchanaburi in Thailand ( Fig. 4 ). If natural selection is driving the echolocation divergence within this population, then genes underlying echolocation frequency should show signs of divergent selection on either side of the area of abrupt echolocation change ( Fig. 4 ). This type of divergent selection has been shown in coat colour genes in dark- and light-coloured populations of Peromyscus living on dark and light soil, respectively [26] . The 15 microsatellites from 462 Craseonycteris individuals were tested for selection based on the F st outlier approach [27] . One microsatellite locus (CTC1; arrow in Fig. 5a–c ) showed strong signs of divergent selection when comparing colonies on either side of the area of abrupt echolocation change (Lositan; P <0.001, Fig. 5a,d,e ), but not when comparing colonies within each side (Lositan; P >0.05, Fig. 5b,c ). The identification of CTC1 as being under selection was also recovered when testing for selection using a hierarchical framework integrating population structure ( Supplementary Information ). We then identified the genomic region containing the microsatellite locus under selection, which was located on the 5′-side of the recombination signal–binding protein for immunoglobulin kappa J region ( RBP-J gene; Supplementary Table S6 ). The RBP-J gene has been shown to be involved in hair cell formation in the cochlea [28] , [29] . As bats are using the highest frequencies of all terrestrial mammals, their hearing system and particularly the hair cells in the organ of Corti, where the sound is received and amplified, need to be well adapted [22] . The microsatellite itself is most likely not under selection, but may be linked to parts of the genome that are under selection, and the RBP-J gene may be another candidate 'echolocation' gene, although further investigations are needed to confirm this. 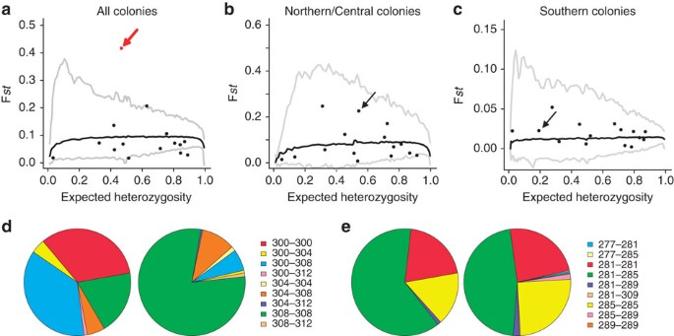Figure 5: Results of Fstoutlier approach detecting microsatellites deviating from model of neutral evolution. Solid back lines represent the average expected distribution under a neutral model, and the grey lines indicate the upper and lower 99% confidence interval for the expected. Each dot represents a microsatellite locus (the locus CTC1 is indicated by an arrow), red dots identifying candidates under positive selection, (a) for all investigated colonies, (b) for colonies North of the area of abrupt echolocation change (colonies A to F), and (c) for colonies South of the area of abrupt echolocation change (colonies G to O). Genotype frequencies are represented for Northern/Central (left) and Southern (right) colonies in Thailand, for two loci, (d) under selection (CTC1) or (e) evolving neutrally (CTC104). Figure 5: Results of F st outlier approach detecting microsatellites deviating from model of neutral evolution. Solid back lines represent the average expected distribution under a neutral model, and the grey lines indicate the upper and lower 99% confidence interval for the expected. Each dot represents a microsatellite locus (the locus CTC1 is indicated by an arrow), red dots identifying candidates under positive selection, ( a ) for all investigated colonies, ( b ) for colonies North of the area of abrupt echolocation change (colonies A to F), and ( c ) for colonies South of the area of abrupt echolocation change (colonies G to O). Genotype frequencies are represented for Northern/Central (left) and Southern (right) colonies in Thailand, for two loci, ( d ) under selection (CTC1) or ( e ) evolving neutrally (CTC104). Full size image Ecological factors driving divergent echolocation From an ecological perspective, the reasons for this sudden change in echolocation peak frequency are not well known. Under an adaptive hypothesis, it would be driven by abiotic or biotic factors [11] . Abiotic factors such as temperature and humidity affect the attenuation of sound (echolocation call) in the air in a frequency-dependant manner, and therefore influence the maximum distance of prey detection [30] , a process that could be responsible for differences in echolocation frequency between populations living in different areas and facing dissimilar climatic conditions [11] . Nevertheless, the resulting interplay of temperature and humidity conditions throughout the Craseonycteris range in Thailand shows little variation, suggesting that attenuation should be constant throughout the range and therefore have a limited role in shaping the echolocation call's frequency ( Fig. 6 ). Furthermore, the observed differences in echolocation frequency result in high sound attenuation values in the Southern colonies (colonies I to O, Fig. 6 ). If the Southern colonies had a peak frequency similar to Northern/Central colonies ( ∼ 74 kHz, colonies A to F), they would benefit from an increased detection distance and the attenuation would be very similar across colonies. Rather, the difference in echolocation frequency seems to render the Southern colonies less-optimal in terms of prey detection distance (for example, increased sound attenuation; Fig. 6 ). Therefore, it seems unlikely that echolocation frequency has changed to keep attenuation constant across the different colonies. 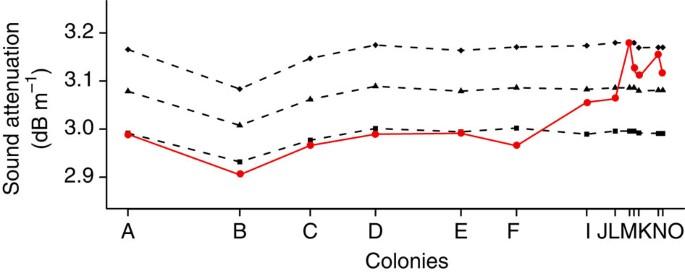Figure 6: Sound attenuation for the different colonies. Sound attenuation is higher for Southern colonies using higher frequencies. The attenuation for the observed frequency (red) shows a higher variability compared with calculated attenuation if colonies had a similar frequency (74 kHz, squares; 75.5 kHz, triangles; 77 kHz, diamonds). Colonies are arranged on theXaxis according to their score at the first axis (explaining 98.9% of the variance) of a principal component analysis on their geographic coordinates (latitude, longitude). Figure 6: Sound attenuation for the different colonies. Sound attenuation is higher for Southern colonies using higher frequencies. The attenuation for the observed frequency (red) shows a higher variability compared with calculated attenuation if colonies had a similar frequency (74 kHz, squares; 75.5 kHz, triangles; 77 kHz, diamonds). Colonies are arranged on the X axis according to their score at the first axis (explaining 98.9% of the variance) of a principal component analysis on their geographic coordinates (latitude, longitude). Full size image Response to different biotic factors (such as interspecific competition) could explain the pattern of echolocation call variation [31] . A shift in peak frequency (character displacement) may act to avoid using the same frequency bandwidth as another small sympatric bat species, Myotis siligorensis . Despite being phylogenetically distant, C. thonglongyai and M. siligorensis produce similar echolocation calls at ∼ 70 kHz (ref. 18 ; Fig. 7 ), are comparable in size, forage in the same habitat and exhibit similar hunting behaviour [18] . This hypothesis would be supported if M. siligorensis was more abundant in the south of Kanchanaburi, where C. thonglongyai has a high echolocation call, than in the North/Centre, where C. thonglongyai peak frequency is lower ( Fig. 4 ). To test this character displacement hypothesis, we visually screened 1,775 recordings from the surrounding areas of 14 caves, where we caught C. thonglongyai . Indeed, in six out of eight sites surveyed in the South, M. siligorensis was recorded multiple times (230/1,327 recordings), whereas in the North/Centre, no individual was recorded at any of the six sites surveyed (0/448 recordings; Fig. 1 ). 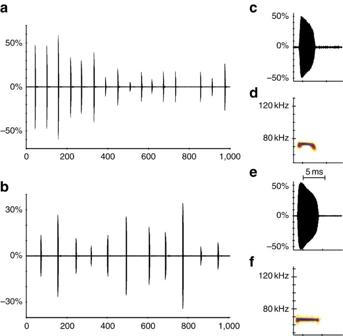Figure 7: Comparison of echolocation calls betweenC. thonglongyaiandM. siligorensis. The calls ofC. thonglongyai(top panels) andM. siligorensis(bottom panels) were recorded from free flying bats in an open environment. The amplitude panelsaandbshow the pattern of calls over a period of 1 s forC. thonglongyai((a), interval between calls=62 ms) andM. siligorensis((b), interval between calls=87 ms). Panelscandeshow in detail the amplitude for one call per species, whereas panelsdandfshow the fast Fourier transformation spectrogram of these same calls. Frequency change over time for one call per species can be seen in the spectrograms. For all panels, theXaxis represents time (in ms). Figure 7: Comparison of echolocation calls between C. thonglongyai and M. siligorensis . The calls of C. thonglongyai (top panels) and M. siligorensis (bottom panels) were recorded from free flying bats in an open environment. The amplitude panels a and b show the pattern of calls over a period of 1 s for C. thonglongyai (( a ), interval between calls=62 ms) and M. siligorensis (( b ), interval between calls=87 ms). Panels c and e show in detail the amplitude for one call per species, whereas panels d and f show the fast Fourier transformation spectrogram of these same calls. Frequency change over time for one call per species can be seen in the spectrograms. For all panels, the X axis represents time (in ms). Full size image The extent of gene flow is of crucial importance during the speciation process; for example, the complete absence of gene flow between two populations of the same species will lead these populations to accumulate genetic differences through time while keeping a pool of complementary genes within each population. The Bateson–Dobzhansky–Muller model [32] , recently supported by empirical evidence [33] , proposes that given enough time, hybrid sterility and inviability will evolve between these two populations due to negative genetic interactions between two or more loci that have accumulated substitutions, ultimately leading to speciation. This process is most likely ongoing between the allopatric Thai and Myanmar populations. The Thai and Myanmar populations of C. thonglongyai are genetically isolated from each other and show marked echolocation differences. Whether these changes in echolocation have had a major role in the separation of the two populations remains difficult to test. The significantly reduced diversity of the Myanmar population suggests that either the population was previously more diverse and went through a bottleneck or that the population originated from the Thai population via a founder effect. It is difficult to rule out the bottleneck hypothesis, but if this scenario was correct, it would mean that the population was severely reduced to a point where all individuals shared the same haplotype. Although not impossible, this scenario seems unlikely. The recent origin of the Myanmar population from the Thai population via a founder effect is more likely and would explain the reduced level of diversity, whereby only a few individuals founded the Myanmar population. Although possible, an active dispersal of a few Craseonycteris from Thailand to Myanmar (200 km) is unlikely given the very short dispersal distance estimated for Craseonycteris (about 2–5 km) and its very localized foraging activity (about 1 km from the colony) [34] . A more plausible scenario would be a 'sweepstakes' dispersal event [35] of a few Craseonycteris via storms, cyclones or typhoons. The winter monsoon winds, blowing from East-South-East to West-North-West, could easily transport Craseonycteris over the 200 km separating the two populations. Episodes of strong winter monsoon winds correspond to orbital periods and have happened every 100-kyr in the past 600-kyr (refs. 36 , 37 ). This 'sweepstakes' event would have been immediately followed by isolation and the absence of gene flow between the two populations. The date of the split was dated between 268,000 and 545,000 years BP, which spans over four periods of high winter monsoon activity [36] . It thus seems that although echolocation differences match perfectly with genetic differences, echolocation probably did not have a role in the separation of the Thai and Myanmar populations. Interestingly, M. siligorensis was captured and/or recorded at all study sites in Myanmar ( Fig. 1 ), further supporting the possible link between the presence of M. siligorensis and high-frequency echolocation calls. The analyses at the population level within Thailand further illuminate the contribution of different factors during the speciation continuum [7] . Even in the best known examples of 'sympatric' speciation, driven by sensory ecology (for example, the Cichlids in Lake Victoria [3] ), it is uncertain whether the variation in sensory traits is the cause or the consequence of the populations' isolation [6] . The quasi-linear distribution of Craseonycteris along the Kwae river valley [16] combined with limited dispersal abilities have shaped a unique system in which to study the contribution of various factors to population structure and gene flow. Within Thailand, isolation by geographic distance seems to be the main factor driving the genetic isolation of populations, a result consistent with recent simulations [38] . If echolocation differences were the primary driver of the populations' isolation, they should explain a much higher percentage of genetic variance and also consistently match the genetic distance, which was not the case. Our results rather support that echolocation differences evolved secondarily in a context of limited gene flow. Limited gene flow can enhance rapid local adaptation [39] and even lead to parapatric speciation in the absence of any environmental variability [38] . We however suggest that in C. thonglongyai , limited gene flow creates the conditions that favour the evolution of echolocation differences via local adaptation and we predict that reinforcement-like selection might drive the speciation process through acoustic isolation limiting mate choice to similar acoustic types [5] , [15] ( Supplementary Note 1 ). Further studies investigating mate-choice preference and survival of individuals in relation to echolocation call frequency are needed to test if this predicted reinforcement-like selection would occur. The 'echolocation' displacement observed could have two functions, which are not necessarily mutually exclusive ( Supplementary Note 2 for further details); species echolocating at different frequencies can in theory detect different sizes of insect prey [40] , thereby, partition food resources, especially if the prey size distribution is skewed towards small prey [41] . However, this hypothesis has received little empirical support in the literature, especially when the echolocation frequency differences between species are less than 10 kHz as in the present case [42] (see ref. 43 ). Alternatively, this character displacement could enable the two species to avoid jamming each other's echolocation system by each having a private bandwidth [44] , and therefore reduce interference competition. In echolocating bats, the onset of the emitted call activates a neuronal gating mechanism that establishes a time window during which pulse-echo pairs are processed for target distance determination [44] . If an echolocation call of a similar frequency is played to an echolocating bat during this time window, the bat is unable to accurately determine target range [45] . Therefore, given the similarity in calls between C. thonglongyai and M. siligorensis , an upward shift in frequency, as seen in the Southern C. thonglongyai population where M. siligorensis is present, could have occurred to avoid acoustic jamming. We note that this idea is consistent with the fact that C. thonglongyai 's calls are also emitted at high frequencies in Myanmar, where M. siligorensis occurs. This work shows that sensory ecology and genetic divergence are associated at the early stage of population differentiation, and that echolocation divergence most likely occurs in a context of limited gene flow, in response to a competitor bat species. We posit that this echolocation divergence may later act to further drive population differentiation within Thailand. Our work highlights the importance of environmental factors (biotic and abiotic) in contributing to population structure and shows the strength of studying the speciation process using both a 'spyglass' and 'magnifying glass' approach. Ongoing studies of these unique Thai and Myanmar populations of C. thonglongyai will provide an opportunity to study the long-term interaction between gene flow and sensory ecology to fully understand the intricacies of the speciation process in nature. Owing to the central role of echolocation in bat biology and its dual role in foraging and communication, further studies using echolocating bats as models to investigate the interplay of sensory ecology, mate choice and gene flow will undeniably advance our understanding of sensory-driven speciation. Echolocation calls Free flying bats were recorded at dusk for 1 h outside the cave's entrance using a D1000X ultrasound detector (Pettersson Elektronik AB) and automatically stored in a memory card (Compaq Flash, SanDisk Ultra II, 1 or 4 GB). A sampling frequency of 384 kHz was used, enabling aliasing-free sounds to be recorded up to 153 kHz. For analysis, calls were processed through a Fast Fourier Transformation (1,024 points, Hanning window, fast Fourier transformations calculated with 90% time overlap; software BatSound version 3.31, Pettersson Elektronik AB). Peak frequency (that is, frequency with most energy) was measured using the function 'Pulse Characteristics Analysis' available in BatSound. The 'mark positioning' was enabled and measurements were visually checked. Each individual's recording contained multiple calls. Our echolocation call data set consisted of 5,650 calls from 376 recordings. To compare the peak frequency between Thailand and Myanmar, we used a generalized linear mixed model via the 'lmer' function implemented in the 'lme' package in R 2.12.0 (ref. 46 ). This model considers the nested structure of individuals within sites and sites within countries. A model with calls nested within individuals was too large to be run; therefore, to remove any potential bias caused by non-independence between calls from the same recording, we generated 10,000 data sets by randomly picking only one call per recording, when performing the generalized linear mixed model. The generalized linear mixed model was performed 10,000 times resulting in10,000 P -values from which we calculated the median. Sample collection and DNA extraction C. thonglongyai of both sexes were sampled from 15 colonies in Thailand ( n =468) and 4 colonies in Myanmar ( n =202; Fig. 1 ). Bats were captured either with a hand-net, while they were roosting during the day, or with mist-nets on emergence at dusk. Bats were placed in cloth bags and immediately released after processing. Two skin biopsies were taken and stored in 200-μl pure ethanol or dried with silica-gel until extraction. DNA was extracted from wing biopsy punches using a modified salt/chloroform extraction protocol [47] that included an additional chloroform/isoamyl alcohol (24/1) step after adding the saturated NaCl solution. DNA samples were used at a final concentration of 2–5 ng · μl −1 ( Supplementary Methods ). Microsatellite genotyping and analysis The 15 microsatellite primers used in this study were specifically developed for C. thonglongyai and were amplified and genotyped following Puechmaille et al . [48] (locus CTD114 not used). To check for genotyping consistency, 10% of samples were amplified and genotyped twice. A total of 670 samples were genotyped for 15 microsatellite loci. Samples were collected on different dates and therefore it was possible that the same individual had been sampled twice. We thus compared multilocus genotypes using GeneCap [49] to identify and remove duplicates from the data set [50] . Out of 670 samples, 11 samples were duplicates (6 in Myanmar and 5 in Thailand), leaving a total of 659 individuals for the analysis (463 and 196 for Thailand and Myanmar, respectively). No departures from Hardy–Weinberg and linkage equilibrium were detected at the colony level after Bonferroni correction using Fstat version 2.9.3.2. For the entire data set, population structure was investigated using the program STRUCTURE version 2.2 (ref. 51 ). We used a burn-in length of 10,000 and a run length of 100,000 without prior population information. The burn-in and run length were chosen after an initial test, whereby we looked at the convergence of the values of summary statistics and consistency between runs. All other parameters were left as by default. Ten independent runs were undertaken for K- values ranging from 1 to 10, reflecting the minimum and maximum number of populations suspected. The number of populations was inferred from the ΔK statistic as developed in Evanno et al . [52] Using the 659 individual genotypes, a phylogenetic tree was constructed by the neighbour-joining method with the Da distance. The tree construction was carried out using the program Populations 1.2.30. Within Thailand (463 individuals), F st and population differentiation were calculated and tested using Genepop v 4.0.6 (ref. 53 ). Mitochondrial DNA and phylogenetic reconstruction A 1,840-bp mitochondrial DNA fragment encompassing the entire Cytb , tRNA Threonine, tRNA Proline and part of the control region was amplified by polymerase chain reaction in three overlapping fragments ( Supplementary Fig. S5 and Supplementary Tables S7 and S8 ). Two NUMTs (nuclear pseudogenes) were also amplified and used in the phylogenetic analysis. Using the mitochondrial DNA and the two NUMTs, phylogenetic reconstruction was undertaken using the Bayesian inference in BEAST [54] ( Supplementary Methods ). Nuclear introns primers, polymerase chain reaction and genotyping Five SNPs were identified on four nuclear introns ( Supplementary Table S8 ), two found on the X chromosome ( BGN and PHKA2 ), the Y chromosome ( SMCY7 ) and one on chromosome 16 for Homo sapiens ( ZP2 ). For these five SNPs, we designed custom TaqMan SNP assays (Applied Biosystems; Supplementary Table S9 ) and screened the 659 individuals ( Supplementary Methods ). Genetic diversity indices To test for differences in genetic diversity between the Thai and Myanmar populations, we grouped colonies into two groups corresponding to Thailand and Myanmar and compared their genetic diversity at the nuclear and mitochondrial level in Fstat version 2.9.3.2. Significance was tested using 10,000 permutations. Samples were randomly allocated to the two groups, and the genetic diversity was calculated for each permutation. The P -value of the test was the proportion of randomized data sets giving a larger value for the genetic index than the observed one (one-sided test). Population history and structure The Thai population's demographic history was examined using the mismatch distribution of 462 mitochondrial DNA sequences [55] . Population structure was analysed using principal component analysis on microsatellite data with R version 2.12.0 (ref. 46 ) using the adegenet package version 1.3-0 (ref. 56 ). Simulations of a spatially expanding population mimicking the expansion of the Thai population were carried out in SPLATCHE [57] , and outputs analysed in Arlequin ver 3.5 (ref. 58 ; via arlecore) and displayed in R 2.12.0 (ref. 46 ). A 100×10 lattice was used, representing the distribution of Craseonycteris along the Kwae River valley [16] . Each deme was considered to be sending migrants to its neighbours at a rate m . Once a deme was colonized, its population size grew following a logistic model with rate r and carrying capacity C . The initial population size was set to 2,000 and the 'AllowSourcePopulationOverflow' parameter was set to '0'. A homogene friction map was used. A set of 12 locations spaced evenly along the 'lat' axis of the lattice (starting at deme 4 and every 8 demes) were sampled for 20 individuals. Sampling was carried out just after the entire lattice was completely filled in. A set of 14 unlinked microsatellite loci with a mutation rate of 5×10 −4 were simulated. On the basis of available information on Craseonycteris colony size [16] , the simulations were run for two values of the carrying capacity C , 100 and 250. For each value of C , 12 combinations of the m (0.1, 0.3, 0.5, 0.7) and r (0.1, 0.3, 0.5) parameters were simulated. One hundred replicates were analysed for each combination of parameters. A simulation was considered to give an isolation by distance pattern similar to the observed, if it contained at least one replicate with a maximal F st comprised between 0.2 and 0.3 and a Mantel r greater than 0.9 ( Supplementary Table S3 ). Causal modelling Causal modelling on resemblance matrices [23] , [24] was used to investigate the combination of factors driving genetic differentiation between colonies and the causal relationships between these factors. Mantel and partial Mantel tests were used within the causal modelling framework to assess the support for all possible organizational models [23] , [24] . All tests were conducted with R version 2.12.0 (ref. 46 ) using the package ecodist [59] version 1.1.4, and significance was assessed with 9,999 permutations ( Supplementary Methods ). Selection tests The 15 microsatellites from 463 individuals were tested for selection based on the F st outlier approach [27] using two models, and island model and a hierarchical island model in LOSITAN [60] and Arlequin [58] version 3.5, respectively ( Supplementary Methods ). Microsatellite CTC1 genomic position Before a Blast search, the microsatellite sequence including the flanking regions (total of 599 nt) was repeatmasked (RepeatMasker version open-3.2.8). Only simple repeats corresponding to the microsatellite motif were identified (from nt 347 to nt 408; TCCA motif). A Blastn search with the default settings and 'word size' set to 7 was used to identify genomic regions similar to the microsatellite locus (CTC1) flanking regions. For the 5′-flanking region (346 nt), the best match ( E -value: 9e−39; coverage=84%, identities=221/302 (73%)) was much better than the second ( E -value: 0.07; coverage=14%, identities=41/51 (80%)) or third match ( E -value: 0.25; coverage=10%, identities=32/37 (86%)). Similarly, for the 3′-flanking region (191 nt), the best match ( E -value: 2e−06; coverage=92%, identities=136/181 (75%)) was much better than the second ( E -value: 0.003; coverage=16%, identities=29/31 (93%)) or third match ( E -value: 0.01; coverage=15%, identities=28/30 (93%)). Both flanking region's best matches were situated on Human chromosome number 4 (GRCh37 reference primary), around 50 kb (53,653 for 3′-flanking region and 52,745 for 5′-flanking region) at 5′ side of the 'recombining binding protein suppressor of hairless isoform 3′, also known as RBP-J ( H. sapiens geneID: 3516; chromosome: 4, location: 4p15.2). As we do not know if there is synteny around RBP-J between C. thonglongyai and H. sapiens , we then used Ensembl to identify potential synteny around RBP-J between H. sapiens and 12 other genomes sequenced at high coverage ( Supplementary Table S6 ). We showed that large syntenic blocks (average=30.2 M) around the RBP-J gene in H. sapiens were also present in all species investigated ( Supplementary Table S6 ). Given the conserved synteny observed in other species investigated, it is therefore likely that microsatellite CTC1 in C. thonglongyai is also in the 5′-side of the RBP-J gene. Accession codes: The data have been deposited in the GenBank database under accession codes GU247601 to GU247751 . How to cite this article: Puechmaille, S.J. et al . The evolution of sensory divergence in the context of limited gene flow in the bumblebee bat. Nat. Commun. 2:573 doi: 10.1038/ncomms1582 (2011).